Topological proximity effect in a topological insulator hybrid It is well known that a topologically protected gapless state appears at an interface between a topological insulator and an ordinary insulator; however, the physics of the interface between a topological insulator and a metal has largely been left unexplored. Here we report a novel phenomenon termed topological proximity effect, which occurs between a metallic ultrathin film and a three-dimensional topological insulator. We study one bilayer of bismuth metal grown on the three-dimensional topological insulator material TlBiSe 2 , and by using spin- and angle-resolved photoemission spectroscopy, we found evidence that the topological Dirac-cone state migrates from the surface of TlBiSe 2 to the attached one-bilayer Bi. We show that such a migration of the topological state occurs as a result of strong spin-dependent hybridization of the wave functions at the interface, which is also supported by our first-principles calculations. This discovery points to a new route to manipulating the topological properties of materials. The topological surface state of three-dimensional topological insulators (3D TIs) is protected by time-reversal symmetry and characterized by a linearly dispersing Dirac-cone energy band with helical spin texture [1] , [2] , [3] , [4] , [5] . This peculiar surface state is a consequence of interfacing TIs with an ordinary insulator, including vacuum. When a hybrid structure of a 3D TI and a superconductor is fabricated, it has been predicted that superconducting proximity effect occurring at the interface would lead to the appearance of two-dimensional (2D) topological superconductivity hosting Majorana fermions [6] . Also, when a 3D TI is in contact with a ferromagnetic insulator, the resulting magnetic proximity effect at the interface leads to the opening of a gap at the Dirac point [7] , [8] , which is prerequisite to realizing topological magnetoelectric effects [9] , [10] . On the other hand, no such exotic phenomena have been discovered for the interface between a TI and a metal; in fact, despite the obvious importance of understanding the TI/metal interface for device applications, there have been only a limited number of experimental studies of such an interface [11] , [12] , [13] , while several theoretical predictions have been made on possible proximity effects occurring in TI heterostuctures involving semiconductor, graphene, metal and normal-insulator interfaces [14] , [15] , [16] , [17] , [18] . To search for nontrivial effects at the TI/metal interface, it would be better if the energy bands in the metal are spin split, because spin-dependent phenomena can be more easily studied in such a metal. In the following, we present spin- and angle-resolved photoemission spectroscopy (ARPES) measurements of the TI/metal interface, and show a novel phenomenon termed topological proximity effect, in which the topological Dirac-cone state migrates from the TI surface to an attached metal film. We have chosen ultrathin (only one-bilayer (1BL) thick) 2D films of Bi metal where the Rashba splitting of the energy bands is strong. Also, one would expect the interface effect to become stronger if the energy states of a TI hybridize more strongly with those in a metal. This consideration led us to choose the ternary chalcogenide TI material TlBiSe 2 (ref. 19 ), in which layers of Tl, Se and Bi are covalently bonded and stacked in the sequence of -Tl-Se-Bi-Se- along the [111] direction ( Fig. 1a ). This material has a nontopological cousin, TlBiS 2 (refs 20 , 21 ), which is useful for making a control experiment. The covalent nature of the interlayer bonding in TlBiX 2 (X=S, Se) would leave dangling bonds on the cleaved surface and cause strong hybridization with deposited metals; this is in contrast to Bi 2 Se 3 or Bi 2 Te 3 , whose surfaces have no dangling bonds and consequently the surface states present just a weak hybridization [11] and no change in the topology [12] when interfaced with Bi. It should be noted that 1BL Bi is structurally unstable in a free-standing form and it can only exist on some substrate; it turned out that TlBiS 2 is a useful non-invasive substrate for 1BL Bi to identify the pristine Bi-derived bands, because of its nontopological nature and the resulting absence of any surface state [20] , [21] . We have traced the variation of the electronic states upon depositing Bi on TlBiX 2 , and our core-level analysis suggests that the Bi atoms first passivate the dangling bonds on the cleaved surface and then start to grow layer by layer ( Supplementary Figs 1 and 2 ; Supplementary Notes 1 and 2 ). 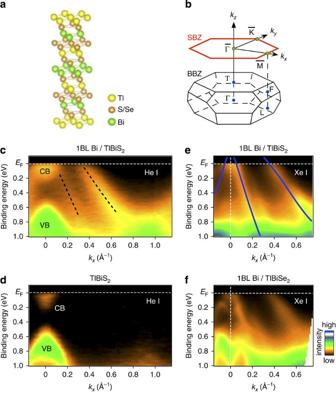Figure 1: Electronic structure of one-bilayer Bi on TlBiS2. (a) Crystal structure of TlBi(S,Se)2. (b) Surface and bulk Brillouin zone (SBZ and BBZ respectively) of TlBiX2(X=S, Se). (c,d) Comparison of the near-EFARPES intensity between 1BL Bi/TlBiS2and pristine TlBiS2measured along the(kx) cut with the He-I photons (hν=21.218 eV) atT=30 K. CB and VB denote the bulk conduction and valence bands of TlBiS2, respectively. (e,f) ARPES intensity around thepoint measured with the Xe-I photons (hν=8.437 eV) for 1BL Bi on nontopological TlBiS2and on topological TlBiSe2, respectively. Calculated band structure for free-standing 1BL Bi is overlaid inewith an upward energy shift of ~0.4 eV, which takes into account the heavily hole-doped nature of the Bi film due to charge transfer to the TlBiX2substrate. Figure 1: Electronic structure of one-bilayer Bi on TlBiS 2 . ( a ) Crystal structure of TlBi(S,Se) 2 . ( b ) Surface and bulk Brillouin zone (SBZ and BBZ respectively) of TlBiX 2 (X=S, Se). ( c , d ) Comparison of the near- E F ARPES intensity between 1BL Bi/TlBiS 2 and pristine TlBiS 2 measured along the ( k x ) cut with the He-I photons ( hν =21.218 eV) at T =30 K. CB and VB denote the bulk conduction and valence bands of TlBiS 2 , respectively. ( e , f ) ARPES intensity around the point measured with the Xe-I photons ( hν =8.437 eV) for 1BL Bi on nontopological TlBiS 2 and on topological TlBiSe 2 , respectively. Calculated band structure for free-standing 1BL Bi is overlaid in e with an upward energy shift of ~0.4 eV, which takes into account the heavily hole-doped nature of the Bi film due to charge transfer to the TlBiX 2 substrate. Full size image Rashba splitting of 1BL Bi/TlBiS 2 Let us start by presenting our control experiment on Bi/TlBiS 2 hybrid. As one can see in the ARPES data along the cut (the bulk and surface Brillouin zones and their high-symmetry points are depicted in Fig. 1b ), the Bi deposition creates a couple of hole-like bands centred at the point (dashed curves in Fig. 1c ) superimposed on the bulk bands of the pristine TlBiS 2 ( Fig. 1d ). These bands are attributed to the quantum-well states (quantized bulk bands) of Bi because of their 2D nature, which can be inferred from the photon-energy invariance of the band location for the He-I ( hν =21.218 eV) and Xe-I ( hν =8.437 eV) photons ( Fig. 1c,e ). Successful fabrication of 1BL Bi films can be judged from the agreement between the observed quantum-well states (called Bi bands hereafter) and the calculated band structure for free-standing 1BL Bi (blue line in Fig. 1e ). When closely examined, the Bi bands present evidence for Rashba spin-splitting. As visualized in the second-derivative ARPES intensity plot of the energy distribution curves (EDCs) along the cut for the 1BL Bi/TlBiS 2 hybrid in Fig. 2a , a pair of dispersions can be found for each of the large and small hole-like bands; we emphasize that the band dispersions determined from the peak positions in the momentum distribution curves (MDCs) by numerical fittings ( Supplementary Fig. 3 and Supplementary Note 3 ), shown with white dots in Fig. 2a , agree with the second-derivative peaks in the EDCs, so the splitting of the bands is a robust observation. Those four bands each form a Fermi surface (labelled LO, LI, SO and SI, standing for ‘large outer’ etc.) as shown in Fig. 2b , in which the two large pockets (LI and LO) exhibit a sizable warping. 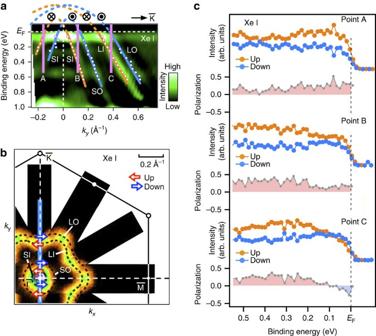Figure 2: Rashba spin-splitting of one-bilayer Bi on TlBiS2. (a) Second-derivative intensity plot of the EDCs for 1BL Bi/TlBiS2hybrid measured along the(ky) cut, together with the location of thekpoints (solid lines) where the spin-resolved ARPES measurements were performed (points A–C). White dots are the peak position of the MDCs estimated by numerical fittings, and dashed orange and blue curves are guides to the eyes to trace the band dispersion. LO, LI, SO and SI represent the large outer, large inner, small outer and small inner hole-like bands, respectively. The direction of the spin-polarization vector for each band is also indicated. (b) ARPES intensity mapping atEFin a 2D wave-vector plane obtained with the Xe-I photons for 1BL Bi/TlBiS2hybrid; this intensity is obtained by integrating the spectra within ±10 meV ofEF. Definitions of the up/down-spin vectors and the experimentally determined spin direction for each Fermi surface are also indicated. (c) Spin-resolved EDCs and corresponding energy dependence of the spin polarization at representativekpoints (A–C) shown ina. Figure 2: Rashba spin-splitting of one-bilayer Bi on TlBiS 2 . ( a ) Second-derivative intensity plot of the EDCs for 1BL Bi/TlBiS 2 hybrid measured along the ( k y ) cut, together with the location of the k points (solid lines) where the spin-resolved ARPES measurements were performed (points A–C). White dots are the peak position of the MDCs estimated by numerical fittings, and dashed orange and blue curves are guides to the eyes to trace the band dispersion. LO, LI, SO and SI represent the large outer, large inner, small outer and small inner hole-like bands, respectively. The direction of the spin-polarization vector for each band is also indicated. ( b ) ARPES intensity mapping at E F in a 2D wave-vector plane obtained with the Xe-I photons for 1BL Bi/TlBiS 2 hybrid; this intensity is obtained by integrating the spectra within ±10 meV of E F . Definitions of the up/down-spin vectors and the experimentally determined spin direction for each Fermi surface are also indicated. ( c ) Spin-resolved EDCs and corresponding energy dependence of the spin polarization at representative k points (A–C) shown in a . Full size image We have investigated the in-plane spin polarization by performing spin-resolved ARPES measurements at three representative k points, A, B and C, shown in Fig. 2a . As one can see in the top part of Fig. 2c , the spin-resolved EDCs at point A (where the SO branch is located near E F ; see Fig. 2a ) demonstrate that the up-spin component is dominant, and consequently the spin polarization is positive. Similarly, the up-spin component is more prominent at point B (where the SI branch is located at ~0.4 eV). At point C, on the other hand, a sign reversal in the spin polarization is observed near E F , and this is due to the contribution from the near- E F LO band, while the contribution of the LI band (located at ~0.4 eV) causes a positive spin polarization at higher binding energy; the smallness of the spin polarization for the LO band is probably related to the suppression of photoelectron intensity due to the matrix-element effect (although we have performed measurements at other k points around point C, it was difficult to observe the negative spin polarization at energies away from E F , probably because of the strong intensity smearing of the LO and SO bands). These results establish that the four Bi bands are spin nondegenerate, and therefore they are most likely forming Rashba-split Kramers pairs (the Rashba splitting is also reproduced by first-principles calculations, as detailed later); the spin texture inferred from our spin-resolved ARPES is shown in Fig. 2a,b . The Rashba splitting is likely triggered by an electrostatic potential normal to the surface plane for vacuum/1BL Bi/TlBiS 2 , which breaks space-inversion symmetry. Topological proximity effect in 1BL Bi/TlBiSe 2 Having understood the Bi bands from our control experiment, we now discuss the topological insulator hybrid, 1BL Bi/TlBiSe 2 . One may expect a simple superposition of the Bi bands and the topological Dirac-cone states of TlBiSe 2 , like in 1BL Bi on Bi 2 Te 3 (ref. 11 ). However, stronger hybridization due to the dangling bonds on TlBiX 2 leads to a highly nontrivial band structure. 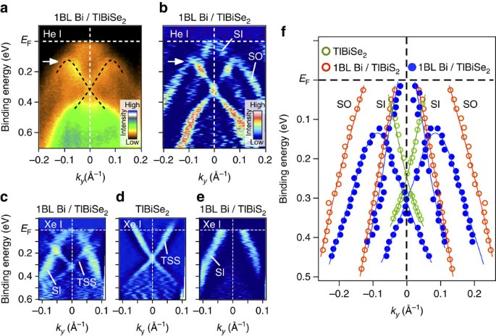Figure 3: Hybridization of topological Dirac-cone and Rashba states. (a,b) ARPES intensity and second-derivative intensity plots of the MDCs, respectively, for 1BL Bi/TlBiSe2hybrid around thepoint obtained with the He-I photons. Black dashed curves inaare guides to the eyes to trace the X-shaped band. White arrow indicates the top of the dispersion for this band. The Bi bands inbare more clearly resolved than those inFig. 2adue to the difference in the derivative variables (that is, d2A/dk2versus d2A/dE2), andnotdue to the difference in the substrates (TlBiS2versus TlBiSe2). (c–e) Second-derivative intensity plots obtained with the Xe-I photons for 1BL Bi/TlBiSe2hybrid, pristine TlBiSe2and 1BL Bi/TlBiS2hybrid, respectively. (f) Experimental band dispersions extracted from the peak positions of the MDCs forb–e. Figure 3a displays the near- E F ARPES intensity around the point measured with the He-I photons, which basically signifies an X-shaped Dirac-cone-like state inside the two Bi bands, SI and SO (the data for a wider energy and momentum range are shown in Fig. 1f ). Obviously, the upper branch of the X-shaped band does not reach E F but exhibits an unusual dispersing-back behaviour with the top of the dispersion at around the intersection with the SO band (white arrow); this situation is better visualized in the second-derivative image of the MDCs in Fig. 3b and the extracted band dispersion in Fig. 3f . One can see that the X-shaped band originates from the topological Dirac-cone state in TlBiSe 2 because (i) it has a 2D nature as confirmed by the hν -invariance ( Fig. 3c ), (ii) its dispersion around the point is similar to that observed in pristine TlBiSe 2 ( Fig. 3d ) and (iii) the X-shaped band is absent in the 1BL Bi/TlBiS 2 hybrid ( Fig. 3e ). Figure 3: Hybridization of topological Dirac-cone and Rashba states. ( a , b ) ARPES intensity and second-derivative intensity plots of the MDCs, respectively, for 1BL Bi/TlBiSe 2 hybrid around the point obtained with the He-I photons. Black dashed curves in a are guides to the eyes to trace the X-shaped band. White arrow indicates the top of the dispersion for this band. The Bi bands in b are more clearly resolved than those in Fig. 2a due to the difference in the derivative variables (that is, d 2 A /d k 2 versus d 2 A /d E 2 ), and not due to the difference in the substrates (TlBiS 2 versus TlBiSe 2 ). ( c – e ) Second-derivative intensity plots obtained with the Xe-I photons for 1BL Bi/TlBiSe 2 hybrid, pristine TlBiSe 2 and 1BL Bi/TlBiS 2 hybrid, respectively. ( f ) Experimental band dispersions extracted from the peak positions of the MDCs for b – e . Full size image We speculate that the observed modulation of the X-shaped band is caused by the strong hybridization through the interface between the upper branch of the Dirac-cone surface state of TlBiSe 2 and the SO band of Bi, as schematically illustrated in Fig. 4a . It is important to recognize that, for such a hybridization to take place, the spin eigenvalue of the two states must agree with each other. In this respect, the upper Dirac cone and the SO band have the same clockwise-rotating spin texture, and hence they can hybridize. This causes the resulting X-shaped band to display a dispersing-back behaviour and, simultaneously, the portion of the SO band near the point is pushed up into the unoccupied region (see right panel of Fig. 4a ). Also, this spin matching argument naturally explains the absence of hybridization between the upper Dirac cone and the SI band seen in Fig. 3b,c . As a result of this spin-dictated hybridization, two new types of bands emerge as shown in the right panel of Fig. 4a : (i) Rashba-split bands of hole character, whose Kramers point was the original Dirac point of TlBiSe 2 and (ii) topological Dirac-cone band (thick curves) whose Dirac point was the original Kramers point of the Rashba-split Bi bands (SO and SI) located above E F . 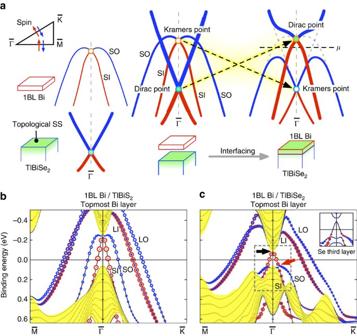Figure 4: Switching between topological Dirac-cone and Rashba states. (a) Schematic illustration of the hybridization between the Rashba-split Bi bands and the topological surface state (SS) of TlBiSe2. Horizontal dashed line in the right panel indicates the location of the chemical potential (μ) in our sample. Blue (red) curves indicate the clockwise- (anticlockwise-) rotating spin texture. (b,c) Calculated band structure for the slab of 1BL Bi on TlBiS2and TlBiSe2, respectively. Spin texture is indicated by circles overlaid on the band dispersion whose colour (blue/red) and radius represent the spin component (clockwise/anticlockwise rotation) and the spin-dependentp-orbital weight at the topmost Bi layer, respectively. Projection of the bulk bands of TlBi(S/Se)2is shown by yellow shade. Black and red arrows incindicate the positions of the Dirac point and the crossing between the Dirac cone and the SO band, respectively. The area enclosed by a rectangle around thepoint incroughly corresponds to the energy region of the schematic band diagram ina. Inset tocshows the calculated band structure for the Se third layer around the Dirac cone, highlighting its small orbital weight in the surface state (circles are negligibly small in this scale). Figure 4: Switching between topological Dirac-cone and Rashba states. ( a ) Schematic illustration of the hybridization between the Rashba-split Bi bands and the topological surface state (SS) of TlBiSe 2 . Horizontal dashed line in the right panel indicates the location of the chemical potential ( μ ) in our sample. Blue (red) curves indicate the clockwise- (anticlockwise-) rotating spin texture. ( b , c ) Calculated band structure for the slab of 1BL Bi on TlBiS 2 and TlBiSe 2 , respectively. Spin texture is indicated by circles overlaid on the band dispersion whose colour (blue/red) and radius represent the spin component (clockwise/anticlockwise rotation) and the spin-dependent p -orbital weight at the topmost Bi layer, respectively. Projection of the bulk bands of TlBi(S/Se) 2 is shown by yellow shade. Black and red arrows in c indicate the positions of the Dirac point and the crossing between the Dirac cone and the SO band, respectively. The area enclosed by a rectangle around the point in c roughly corresponds to the energy region of the schematic band diagram in a . Inset to c shows the calculated band structure for the Se third layer around the Dirac cone, highlighting its small orbital weight in the surface state (circles are negligibly small in this scale). Full size image Band calculations of 1BL Bi on TlBiS 2 and TlBiSe 2 Our first-principles band structure calculations for model crystals of 1BL Bi on TlBiS 2 and TlBiSe 2 ( Fig. 4b,c ; see Supplementary Fig. 4 and Supplementary Note 4 for details) strongly supports the existence of Rashba-split Bi bands as well as the band diagram speculated above. As shown in Fig. 4b , the calculated band structure for 1BL Bi/TlBiS 2 reproduces many important aspects of the experimental data in Fig. 2 . First, we identify spin-split Bi-derived hole-like bands corresponding to the LO, LI, SO and SI bands in the experiment. Remarkably, the spin texture (clockwise or anticlockwise rotation) for all of these bands is identical to the ARPES data on 1BL Bi/TlBiS 2 (thanks to a small overlap of the Bi bands with the bulk-band projection of TlBiS 2 , the Bi band largely keeps the free-standing-like dispersion in a wide range of the k space). Similar Rashba-split bands are also recognized in the calculated band structure of 1BL Bi/TlBiSe 2 ( Fig. 4c ), although the band structure around the point shows some characteristic differences from the TlBiS 2 hybrid, owing to the hybridization between the Bi bands and the topological Dirac-cone states of TlBiSe 2 . Second, an extremely hole-doped nature of the Bi bands (chemical potential shift of ~0.4 eV) is also reproduced by the calculation in both 1BL Bi/TlBiS 2 and 1BL Bi/TlBiSe 2 , as a consequence of strong hybridization and resulting band repulsion between the S/Se and Bi states due to covalent bonding (note that the predicted 2D TI nature of 1BL Bi and its semiconducting property [22] would not have a role in the electronic states near E F owing to a complete mismatch of the band gaps between 1BL Bi and TlBi(S/Se) 2 , and the physics is essentially that of a metal/insulator heterostructure). Third, in 1BL Bi/TlBiSe 2 ( Fig. 4c ), we recognize a new lower Dirac cone whose Dirac point (black arrow) is located at slightly above E F in the calculation, in agreement with the location of the new Dirac cone expected from ARPES; note that this lower Dirac cone and the SO band intersects without strong hybridization (red arrow), confirming the spin-dictated hybridization. It is noted that while the upper Dirac cone is not visible in this calculation because it is buried in the bulk-band projection (the calculation underestimates the bulk-band gap (~0.1 eV as opposed to ~0.35 eV in the experiment [19] ) due to the well-known limitation of the density functional theory), the lower Dirac cone must connect to an upper branch exactly at the point to produce a full Dirac-cone dispersion, due to its spin nondegenerate nature and the requirement of Kramers degeneracy; in other words, the spin-nondegenerate nature of the SI band and the time-reversal symmetry guarantees the existence of the upper Dirac cone. The SO band which forms the Kramers pair with the SI band in 1BL Bi/TlBiS 2 ( Fig. 4b ) is not responsible for this band connection, since it sinks below E F in 1BL Bi/TlBiSe 2 ( Fig. 4c ). For dispersions below E F , by taking into account the calculated spin helical texture of the SO band and the former lower Dirac cone of the TlBiSe 2 surface state, the existence of the new Kramers point is also assured in 1BL Bi/TlBiSe 2 , even though it is buried in the bulk-band projection in the calculation. It should be noted that the calculated Dirac cone above E F in 1BL Bi/TlBiSe 2 has a dominant contribution from the p orbital of topmost and second Bi layers (85% of total weight; nearly equal contribution from these two layers), suggesting that it is of 1BL-Bi origin and is migrated from the surface of TlBiSe 2 as a result of strong hybridization; this phenomenon may be called a topological proximity effect. Intriguingly, the calculated surface/interface states have an odd number of band crossings in the bulk-band-gap region between two time-reversal-invariant momenta and irrespective of the position of the chemical potential, as opposed to an even number of crossings in 1BL Bi/TlBiS 2 , indicating that the 1BL Bi/TlBiSe 2 hybrid system maintains the topologically nontrivial nature unlike the TlBiS 2 hybrid. This can also be confirmed by counting of experimental band crossings in Figs 2a and 4a . We emphasize that a key ingredient for realizing the present topological proximity effect is to contact a TI with a quasi-2D metal thin film, rather than a 3D bulk metal; in this respect, it may be conceived as a manipulation of the boundary condition for the TI. Besides, the topological proximity effect would not be peculiar to a strongly spin–orbit-coupled metal like Bi, but it would occur for a wider range of metals as suggested in a pioneering theoretical study of proximity effects in semiconductor/TI heterostructures [15] . Fabrications of metal thin films on TIs with various film thickness and their characterizations via spin-resolved ARPES would be particularly useful for studying the topological proximity effect. Topological proximity effect may also have some relevance to applications. For example, it may be possible to enhance the performance of a metallic spintronic material (for example, to generate highly-conducting channel [18] ) by giving it the blessed property of topological protection. Also, fabrication of topologically protected spin-plasmon devices [23] by patterning Rashba metals on the surface of TIs may be conceivable. On the fundamental side, the topological proximity effect is the first step towards understanding the peculiarities of the metal-film/TI interface. Extending the spin-resolved ARPES technique to other TI heterostructures would prove useful for testing theoretical proposals of interesting proximity effects in a variety of TI hetersotructures [14] , [15] , [16] , [17] , [18] . Sample preparation High-quality single crystals of TlBiSe 2 and TlBiS 2 were grown by a modified Bridgman method [20] . To prepare the Bi film, we first cleaved the TlBiSe 2 or TlBiS 2 crystals to obtain a shiny mirror-like surface, and then deposited Bi atoms at room temperature in ultrahigh vacuum of 1 × 10 −10 Torr. The 1 × 1 surface structure originating from Bi was confirmed by the low-energy electron diffraction measurement. The film thickness was controlled by the deposition time at a constant deposition rate. The actual thickness was estimated by a quartz-oscillator thickness monitor and also from a comparison of the ARPES-derived band dispersion with the band-structure calculations for free-standing multi-layer Bi [24] , [25] , [26] . ARPES experiments ARPES measurements were performed with the MBS-A1 electron analyser equipped with high-intensity He and Xe plasma discharge lamps [27] without breaking the vacuum after the Bi film was grown. We used the He-Iα resonance line ( hν =21.218 eV) and one of the Xe-I lines ( hν =8.437 eV) to excite photoelectrons. The energy resolution for the regular and spin-resolved ARPES measurements was set at 6–20 and 40 meV, respectively. The sample temperature was kept at 30 K during the measurements. We used the Sherman function value of 0.07 to obtain spin-resolved ARPES data. How to cite this article: Shoman, T. et al . Topological proximity effect in a topological insulator hybrid. Nat. Commun. 6:6547 doi: 10.1038/ncomms7547 (2015).